Paired oxygen isotope records reveal modern North American atmospheric dynamics during the Holocene The Pacific North American (PNA) teleconnection has a strong influence on North American climate. Instrumental records and century-scale reconstructions indicate an accelerating tendency towards the positive PNA state since the mid-1850s, but much less is known about long-term PNA variability. Here we reconstruct PNA-like climate variability during the mid- and late Holocene using paired oxygen isotope records from two regions in North America with robust, anticorrelated isotopic response to the modern PNA. We identify mean states of more negative and positive PNA-like climate during the mid- and late Holocene, respectively. Superimposed on the secular change between states is a robust, quasi-200-year oscillation, which we associate with the de Vries solar cycle. These findings suggest the persistence of PNA-like climate variability throughout the mid- and late Holocene, provide evidence for modulation of PNA over multiple timescales and may help researchers de-convolve PNA pattern variation from other factors reflected in palaeorecords. Large-scale teleconnections have a significant influence on regional weather and climate [1] . At mid-latitudes in the North Pacific and North American sectors, the Pacific North American (PNA) pattern, which exhibits strong interannual variability and interacts with other climate oscillations and forcings to produce multidecadal [2] , [3] variability, represents the most prominent mode of atmospheric oscillation. The PNA is represented as a standardized index derived from North Pacific and North American mid-tropospheric geopotential height anomalies [1] , with positive PNA (PNA+) conditions associated with enhanced ridge and trough structure and meridional flows over North America and negative PNA (PNA−) with more uniform pressure fields and stronger zonal flows. Similar spatial signatures of pressure and precipitation fields associated with interdecadal or century-scale variability may be described as PNA-like inasmuch as they reflect common, coordinated changes in the atmospheric circulation, but may arise from distinct dynamical mechanisms. PNA is associated with variation in the direction and strength of the prevailing circulation and storm tracks, affecting moisture sources, temperature, precipitation amounts and isotopic composition ( δ 2 H and δ 18 O), mountain snowpack and lake levels across North America [2] , [4] , [5] , [6] . The PNA is most strongly expressed in winter, but can affect climate throughout the year ( Fig. 1 and Supplementary Fig. 1 ). 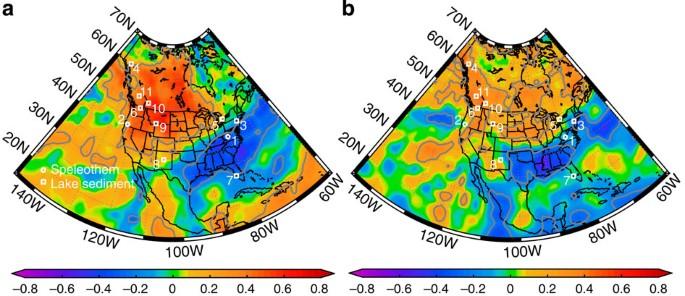Figure 1: Correlations between modelled precipitationδ18O and PNA index. Maps show long-term (1950–2005) correlations between IsoGSM precipitationδ18O and PNA index (Climate Prediction Center) in the North American (NA) continent. (a) Cool season (December–March) correlation. (b) Annual correlation. The areas enclosed by the grey line show significance at theP<0.1 level. Both cool season and annual correlations display a northwest (NW)–southeast (SE) dipolar pattern across the NA continent, with positive correlation in the NW and negative correlation in the SE. Numbers indicate locations mentioned in the text: 1—BCC speleothem14, 2—OCNM speleothem15, 3—Lake Grinnell16, 4—Lake Jellybean10, 5—Crawford Lake29, 6—Castor Lake25, 7—Little Salt Spring24, 8—Estancia Lake23, 9—Crevice Lake26, 10—Dog Lake27, 11—Felker Lake28. Figure 1: Correlations between modelled precipitation δ 18 O and PNA index. Maps show long-term (1950–2005) correlations between IsoGSM precipitation δ 18 O and PNA index (Climate Prediction Center) in the North American (NA) continent. ( a ) Cool season (December–March) correlation. ( b ) Annual correlation. The areas enclosed by the grey line show significance at the P <0.1 level. Both cool season and annual correlations display a northwest (NW)–southeast (SE) dipolar pattern across the NA continent, with positive correlation in the NW and negative correlation in the SE. Numbers indicate locations mentioned in the text: 1—BCC speleothem [14] , 2—OCNM speleothem [15] , 3—Lake Grinnell [16] , 4—Lake Jellybean [10] , 5—Crawford Lake [29] , 6—Castor Lake [25] , 7—Little Salt Spring [24] , 8—Estancia Lake [23] , 9—Crevice Lake [26] , 10—Dog Lake [27] , 11—Felker Lake [28] . Full size image PNA-like variability is driven by internal atmospheric dynamics and external forcing. Instrumental records extending back several decades show an accelerating trend towards PNA+ conditions and a strong modulation of PNA by sea surface temperature (SST) variability [7] , [8] associated with the El Niño/Southern Oscillation (ENSO), Pacific Decadal Oscillation and Atlantic Multidecadal Oscillation. Palaeoclimate studies have adopted PNA as a framework for interpretation of century-scale climate variability in North America, documenting a secular trend towards PNA+ conditions since 1850 and periodic PNA oscillations linked to solar forcing and regional drought [2] , [9] , [10] , [11] , [12] , [13] . Although this work has greatly improved our understanding of the nature of PNA-like climate variability and associated dynamics over annual to multidecadal timescales, long-term variability of the PNA pattern and its relation to external forcing remain poorly known. Here we assess multi-millennial reconstructions demonstrating PNA-like climate variation over a range of timescales. These reconstructions are based on recently documented anti-phase variation in precipitation water isotope ratios in western and eastern North America that is robustly and uniquely associated with variation in PNA-associated circulation patterns [4] , [5] , [6] ( Fig. 1 and Supplementary Fig. 1 ). We compare well-dated, independent palaeoisotope proxy records situated within the western (Oregon Caves National Monument (OCNM) speleothem [14] and Lake Jellybean sediment [10] ; sites 2 and 4 in Fig. 1 and Supplementary Fig. 1 ) and eastern (Buckeye Creek Cave (BCC) speleothem [15] and Lake Grinnell sediment [16] ; sites 1 and 3) regions of isotope/PNA correlation. Each time series consists of carbonate δ 18 O measurements that were re-sampled to a common sampling resolution (47 years for speleothems, 35 years for lake sediments, see Methods) and represents local variation in mid-Holocene (MH) to late-Holocene (LH) precipitation δ 18 O values, likely overprinted by variation in local temperature, humidity and soil or lake water balance. Our results demonstrate anti-phase variability in the eastern and western regions, consistent with the expected expression of variation in the PNA pattern, over both millennial and centennial timescales. These results, supported by analysis of isotope-enabled general circulation model output and independent palaeo-precipitation proxy data, suggest that the PNA pattern may be a persistent pattern of climate system variability that has been modulated by other forcings and feedbacks over timescales of hundreds to thousands of years. Millennial-scale trends Each record ( Fig. 2 ) exhibits substantial isotopic variability through the MH and LH (ranges of values are 1.33‰ at OCNM and 0.90‰ at BCC for speleothem carbonate, and 1.84‰ at Lake Jellybean and 1.66‰ at Lake Grinnell for lake sediment carbonate). Paired values from the re-sampled time series are significantly anticorrelated for each archive ( r =−0.55, P <0.001 and n eff =25 for speleothem and r =−0.13, P <0.1 and n eff =11 for lake sediment, see Methods). Within each region, δ 18 O values of different archives also exhibit statistically significant but positive correlations ( r =0.18, P <0.005 and n eff =15 for the western records, re-sampled at a common 22-year resolution, and r =0.72, P <0.001 and n eff =34 for the east at a 47-year resolution). Data from both lake sediments and speleothems show significant ( P <0.0001) secular change throughout the period of record, with opposing trends for records derived from the western (increasing with time) and eastern (decreasing with time) sites ( Fig. 2 and Supplementary Fig. 2 ). A two-sample t -test shows that the long-term mean values for the MH and LH intervals in each record are significantly different ( P <0.01, see Methods). The anticorrelated change in oxygen isotope ratios in these two regions is consistent with expectations for a shift from a climate state dominated by more PNA−-like circulation conditions during the MH to more PNA+-like conditions during the LH [4] , [5] , [6] . 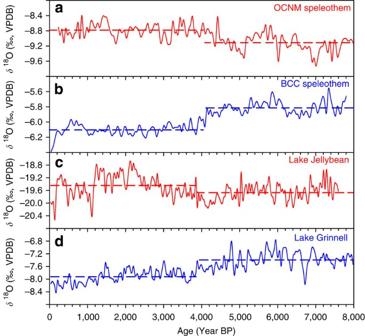Figure 2: Palaeoclimate proxy records from the North American continent. (a) OCNM speleothemδ18O. (b) BCC speleothemδ18O. (c) Lake Jellybean sedimentδ18O. (d) Lake Grinnellδ18O. Red and blue lines denote the records from western and eastern North America, respectively. The dashed lines show the mean values of each record for the MH and LH (for the demarcation of the MH and LH, seeSupplementary Fig. 2). Figure 2: Palaeoclimate proxy records from the North American continent. ( a ) OCNM speleothem δ 18 O. ( b ) BCC speleothem δ 18 O. ( c ) Lake Jellybean sediment δ 18 O. ( d ) Lake Grinnell δ 18 O. Red and blue lines denote the records from western and eastern North America, respectively. The dashed lines show the mean values of each record for the MH and LH (for the demarcation of the MH and LH, see Supplementary Fig. 2 ). Full size image Variation in the individual δ 18 O records has previously been attributed to effects of changing local temperature, precipitation, moisture sources and storm tracks driven by large-scale climate modes [10] , [14] , [15] , [16] . The significant anticorrelated variation identified here for the western and eastern regions suggests that these records are responding to a common, large-scale climatic teleconnection between the regions. We suggest that the inversely correlated component of isotopic change in the western and eastern sites may reflect long-term variability of the mean state of PNA through the Holocene based on the documented association of anti-phase precipitation isotopic variation in these regions with PNA. During the MH, relatively low δ 18 O values in the west coupled with relatively high δ 18 O values in the east are consistent with dominance of a more PNA−-like climate pattern over North America ( Fig. 2 ), supporting enhanced zonal circulation [10] . By contrast, LH isotope records suggest a PNA+-like mean state, characterized by enhanced meridional circulation [17] , [18] with higher δ 18 O values in western North America and lower values in the east. The shift between these states is nearly synchronous with climatic and hydrological changes recorded in a number of different proxies across North America [19] , [20] , [21] , and corresponds temporally with the 4.2–3.9 kyr before present (BP) abrupt climate event documented globally [22] . Our result is supported by independent proxy evidence from a range of sites across the continent. Published MH records suggest drier conditions in the southwestern United States [23] (site 8 in Fig. 1 and Supplementary Fig. 1 ) and Florida [24] (site 7). For the same time interval, wetter conditions are reconstructed in the Pacific Northwest (NW) [25] (site 6), southwestern Montana [26] (site 9) and British Columbia [27] , [28] (sites 10 and 11), and wetter conditions and 18 O-depleted precipitation have been inferred in the Great Lakes region [29] (site 5). This distribution is generally consistent with the pattern of precipitation change associated with the modern PNA− state ( Fig. 3d and Supplementary Fig. 1b ), which features enhanced precipitation across the Pacific NW, Northern Rocky Mountains and upper Midwestern United States, and reduced precipitation in the southwestern and southeastern United States and across the central and southern Great Plains. It is also consistent with expectations [30] , [31] for circulation patterns associated with independently documented negative Pacific Decadal Oscillation and/or La Niña-like patterns in the Pacific [18] , [32] and a positive North Atlantic Oscillation pattern [32] , [33] during the MH. 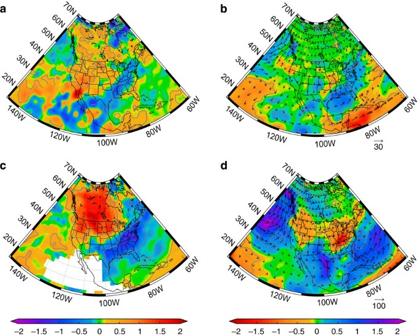Figure 3: Precipitationδ18O and climate field differences. Results are from IsoGSM and show cool season (December–March) differences. (a) Precipitationδ18O (‰, VSMOW) difference between late Holocene (LH) and mid Holocene (MH; LH minus MH). (b) Precipitation (mm day−1) and vertically integrated moisture flux (kg m−1s−1) field difference between LH and MH. (c) Precipitationδ18O (‰, VSMOW) difference between PNA+ and PNA−. (d) Precipitation (mm day−1) and vertically integrated moisture flux (kg m−1s−1) field difference between PNA+ and PNA−. LH simulations are based on a 20-year integration forced with modern SSTs and greenhouse gases and the MH simulation is a 20-year integration using orbital configuration at 6,000 year BP and MH SST forcing (see Methods for the details). The areas enclosed by the grey lines show significant (P<0.1) precipitation and isotope differences. The arrows inbandddenote vertically integrated moisture flux (kg m−1s−1). Figure 3: Precipitation δ 18 O and climate field differences. Results are from IsoGSM and show cool season (December–March) differences. ( a ) Precipitation δ 18 O (‰, VSMOW) difference between late Holocene (LH) and mid Holocene (MH; LH minus MH). ( b ) Precipitation (mm day −1 ) and vertically integrated moisture flux (kg m −1 s −1 ) field difference between LH and MH. ( c ) Precipitation δ 18 O (‰, VSMOW) difference between PNA+ and PNA−. ( d ) Precipitation (mm day −1 ) and vertically integrated moisture flux (kg m −1 s −1 ) field difference between PNA+ and PNA−. LH simulations are based on a 20-year integration forced with modern SSTs and greenhouse gases and the MH simulation is a 20-year integration using orbital configuration at 6,000 year BP and MH SST forcing (see Methods for the details). The areas enclosed by the grey lines show significant ( P <0.1) precipitation and isotope differences. The arrows in b and d denote vertically integrated moisture flux (kg m −1 s −1 ). Full size image General circulation modelling Results from the proxy data are further supported by climate model output from the Isotopes-incorporated Global Spectral Model (IsoGSM [34] ) and the Paleoclimate Modelling Intercomparison Project Phase III archive. We evaluated IsoGSM simulations forced with MH and LH boundary conditions (see Methods), which show a spatially coherent pattern of winter precipitation δ 18 O change across the North American continent ( Fig. 3a ). LH conditions feature higher δ 18 O values in the NW and slightly lower values in the southeast ( Fig. 3a ). Similar patterns of isotope change also exist if this comparison is conducted for annual average values, but with weaker spatial coherence ( Supplementary Fig. 3 ). The IsoGSM results are roughly consistent with results from other isotope-enabled atmospheric (LMDZ-iso [35] ; Supplementary Fig. 4 ) and coupled ocean-atmosphere (ModelE [36] ) models. Comparison of the IsoGSM results with simulations from non-isotope-enabled models included in the Paleoclimate Modelling Intercomparison Project Phase III shows broad congruence in patterns of precipitation change between the MH and LH ( Supplementary Fig. 5 ). Drier conditions dominate across southeastern North America in all models and half of models simulate slightly wetter conditions in the NW (HadGEM2-CC, IsoGSM, MIROC-ESM, MPI-ESM-P and MRI-CGCM3) during the MH, further supporting the robustness of the hydrological changes simulated by IsoGSM. The isotope changes simulated in IsoGSM are associated with enhanced southwesterly moisture flux (delivering vapour more enriched in 18 O) to NW North America and northerly to easterly moisture flux (more depleted in 18 O) to southeast North America during the LH compared with MH ( Fig. 3b ). Despite differences in magnitude, the spatial structure of modelled isotope and climate field differences between LH and MH is similar to that between the PNA+ and PNA− states ( Fig. 3 , Supplementary Fig. 6 ), supporting our interpretation that MH to LH shifts in the proxy records may reflect a change in the mean state of the PNA pattern. Changes in pressure fields between the two modelled Holocene states are similar to those associated with modern PNA, characterized by positive surface pressure anomalies that arc from the Hawaiian Islands over the western interior of North America and negative surface pressure anomalies over the southeastern United States and/or Aleutian Islands during LH ( Supplementary Fig. 7 , except GISS-E2-R). Modelled LH conditions are also characterized by a more negative NAO-like pattern in north Atlantic pressure ( Supplementary Fig. 7 , except CCSM4, HadGEM2-CC and MRI-CGCM3), and a more El Niño-like pattern in the tropical Pacific SSTs (relative to modelled MH conditions; Supplementary Fig. 8 , except GISS-E2-R and HadGEM2-CC), consistent with previous palaeoclimate reconstruction [18] , [33] and modelling [37] , [38] . Centennial-scale variability The oxygen isotope proxy records also exhibit substantial short-term (centennial) variation superimposed on the millennial-scale trends. Cross-spectral analysis for paired speleothem or sediment δ 18 O records from the two regions indicates coherent, statistically significant (>90% confidence) variability at periodicities of 195 years for speleothems and 219 years for lake sediments ( Fig. 4a,b ). Although similar coherent periodicities can also be identified in cross-comparisons of the records from the two regions (that is, speleothem versus lake sediment) these are not statistically significant ( Supplementary Fig. 9 ), perhaps due in part to differences in time averaging and/or resolution of the different archives. Band-pass-filtered δ 18 O records targeting these frequencies show robust ( r =−0.96, P <0.0001 for speleothem and r =−0.95, P <0.0001 for lake sediment) anti-phase oscillations, consistent with expected response to PNA pattern variation ( Fig. 4c,d and Supplementary Fig. 10 ). Filtered records from all sites exhibit similar patterns of amplitude modulation throughout the period of record. Although the period of these variations approaches the limits of uncertainty associated with the proxy record age models, the common signal in all four records, in terms of both frequency and amplitude, suggests that they are responding to common, large-scale forcing. Furthermore, age model errors could only explain the anti-phase, PNA-like oscillations recorded by both proxy pairs in the event that there were systematic biases producing a common phase-shift in both lacustrine and speleothem records, an unlikely occurrence. Comparison of the δ 18 O records from the eastern sites with an independently reconstructed, 1,000-year PNA index [12] reveals strong coherence of phase and amplitude variations within the ~200-year periodicity domain (inset panels in Fig. 4c,d ), further supporting the identification and extrapolation of PNA variability in this frequency domain throughout the MH and LH. 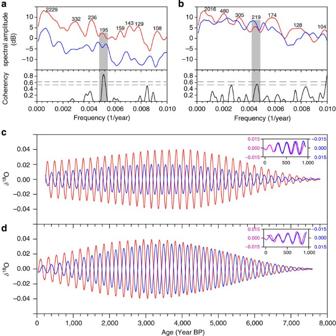Figure 4: Spectral analysis of speleothem and lake sedimentδ18O records. (a,b) Power and coherency spectra for (a) OCNM (red) and BCC (blue) Speleothemδ18O records and (b) Lake Jellybean (red) and Lake Grinnell (blue) sedimentδ18O records. The cross-spectral analysis was performed using computer package SPECTRUM48(see Methods). Periods of the main spectral peaks are labelled. The horizontal dashed lines indicate significance at the 90 and 95% level in the coherence spectra. Grey bars denote significantly strong coherence between paired proxyδ18O records. (c) Paired speleothemδ18O time series after 195±5 year band-pass filtering. (d) Paired lake sedimentδ18O time series after 219±5 year band-pass filtering. Insets incanddare the comparisons of BCC speleothem and Lake Grinnellδ18O records with independently reconstructed PNA index values12(pink line) filtered in the 200±5 year periodicity domain. Note that theδ18O records are inverted to express their anticorrelation with the PNA index. All filtering used a third-order Butterworth band-pass filter. Figure 4: Spectral analysis of speleothem and lake sediment δ 18 O records. ( a , b ) Power and coherency spectra for ( a ) OCNM (red) and BCC (blue) Speleothem δ 18 O records and ( b ) Lake Jellybean (red) and Lake Grinnell (blue) sediment δ 18 O records. The cross-spectral analysis was performed using computer package SPECTRUM [48] (see Methods). Periods of the main spectral peaks are labelled. The horizontal dashed lines indicate significance at the 90 and 95% level in the coherence spectra. Grey bars denote significantly strong coherence between paired proxy δ 18 O records. ( c ) Paired speleothem δ 18 O time series after 195±5 year band-pass filtering. ( d ) Paired lake sediment δ 18 O time series after 219±5 year band-pass filtering. Insets in c and d are the comparisons of BCC speleothem and Lake Grinnell δ 18 O records with independently reconstructed PNA index values [12] (pink line) filtered in the 200±5 year periodicity domain. Note that the δ 18 O records are inverted to express their anticorrelation with the PNA index. All filtering used a third-order Butterworth band-pass filter. Full size image Our results identify similar, spatially structured changes in North American hydroclimate occurring on two different timescales during the Holocene. The pattern of change in isotopic records, climate model simulations and independent proxy data are similar to that associated with modern PNA, suggesting that these records may reflect a common pattern of atmospheric variability reminiscent of, or involving, a change in the mean state of PNA. If so, PNA may represent a persistent pattern of climate system variability throughout the MH to LH, which was modulated by changes in forcing and/or interaction with other dynamical modes over a range of timescales. The transition between the MH and LH is characterized by a substantial change in insolation that affected many parts of the climate system [32] . PNA-like changes in North American climate at this time may reflect the influence of orbitally driven meridional migration of the intertropical convergence zone (ITCZ) and ENSO. The MH to LH decrease in summer/annual insolation has been associated with a southward shift of the ITCZ [39] . Southward displacement of the ITCZ induces a PNA-like extratropical atmospheric response [40] , with a barotropic ridge over the Rocky Mountains accompanied by a deepened trough (a southward shift of the polar jet) in southeastern North America in winter. This would lead to drier conditions in northwestern North America and wetter conditions in the southeastern United States during the LH ( Supplementary Fig. 5 ). This PNA-like response is further amplified by a warm LH eastern tropical Pacific SST (as during El Niño; Supplementary Fig. 8 ) that can produce enhanced Rossby wave propagation from the tropical Pacific, directly exciting the PNA pattern [41] . Centennial-scale North American climate variability during the Holocene has previously been linked to variations in solar radiation [42] . The 195- and 219-year periodicities identified and associated with modulation of palaeo-PNA variability here are similar to that of the 210-year de Vries (Suess) solar cycle [43] , which may suggest a persistent link between PNA-associated North American climate changes and solar variability during the MH and LH. Previous studies have demonstrated that variation in solar ultraviolet radiation can lead to shifts in regional atmospheric circulation patterns and the polar jet through heating and ozone chemistry in the middle atmosphere [44] . North American circulation patterns for low and high solar activity winters during the period of instrumental record show strong associations with PNA+ and PNA− circulation patterns, respectively [45] ( Supplementary Fig. 11 ). A recent 275-year PNA reconstruction further supports this association, with two prominent solar minima (Dalton and Damon) being characterized by strong PNA+ conditions [2] . Hydroclimatic variability in continental North America is closely linked to the large-scale circulation, and a large number of studies have previously related regional palaeoclimatic change to storm tracks and moisture transport [10] , [11] , [12] , [13] , [14] , [15] , [17] , [25] , [29] . Our work suggests strong, continental-scale coherency in these changes at centennial to millennial scales throughout the past 8,000 years. The association of MH to LH isotopic and climatic variability with PNA-like shifts in atmospheric circulation suggests that the PNA pattern was a persistent feature of the North American climate. Given demonstrated links between other major climatic modes and the PNA pattern, modulation of PNA variation offers a unifying and consistent framework for translating large-scale climate system trends (for example, MH to LH shifts in ENSO [18] , [32] ) and variability (for example, in response to solar cycles [43] , [44] ) into regionally coherent climatic change across North America. This framework could be further tested as transient climate model simulations spanning this period of Earth history become available. The proposed associations may provide an indication of the spatial structure of future continental hydroclimatic impacts expected under shifting climatic regimes (for example, Fig. 3 ). In addition, our work indicates systematic, regional variation in moisture sources and precipitation δ 18 O values throughout the MH to LH, and recognition of these patterns will be important for de-convolving these large-scale changes from variation in other regional or local climatic variables reflected in palaeoclimate proxy archives. Selection of palaeoclimate proxy records Two pairs of palaeoclimate proxy records were selected for analysis, including speleothem records from West Virginia (BCC) and Oregon (OCNM) and lake sediment records from New Jersey (Lake Grinnell) and Yukon (Lake Jellybean). With the exception of Lake Grinnell, the records were retrieved from the NOAA World Data Center for Paleoclimatology ( http://www.ncdc.noaa.gov/paleo/data.html ). The records were chosen based on two primary selection criteria: proximity of the study site relative to the two poles of correlation between modern isotopes in precipitation and PNA index, and high temporal resolution (average sampling interval of 50 years or better) throughout the MH and LH. Age model and re-sampling of time series data Age models for all sites are derived from the original data source and are fully described in the primary references. The BBC age model was based on linear interpolation between U/Th ages for each speleothem. Average analytical uncertainty (2 σ ) for the individual age determinations was 49 years [15] . The OCNM speleothem age model was derived from 29 high-precision U/Th dates using Markov Chain Monte–Carlo sampling and Bayesian statistics [14] . The average uncertainty (2 σ ) for the individual age determinations through the period of record used here was 140 years. The Lake Grinnell sediment core was dated using seven accelerator mass spectrometry 14 C determinations on terrestrial plant macrofossils, with an average uncertainty (2 σ , calibrated age) throughout the period of record used here of 49 years [16] . Ages were assigned using a fourth-order polynomial curve fit to these data, with a fixed surface age (−55 cal year BP=2005 AD). The chronology of the Lake Jellybean sediment core was determined based primarily on seven accelerator mass spectrometry 14 C measurements of terrestrial macrofossils and pollen, supported by 210 Pb and 137 Cs data from shallow sediments and identification of an independently dated ash layer [10] . Uncertainty (1 σ ) in the calibrated radiocarbon ages varies from 80 to 157 years (average=120 years). All ages discussed in this paper are reported using calendar years BP, where present is defined as 1950 AD. Ages post-dating 1950 are reported as negative. For speleothem records, BCC is derived from records from three speleothems: BCC2, BCC4 and BCC6, with an average time resolution of 35, 46 and 47 years, respectively. The three raw BBC speleothem chronologies were combined to yield a composite representative of the underlying climate variability. To this end, each speleothem record was re-sampled at common, 47-year intervals, using linear interpolation between data points. A composite time series was calculated by averaging values from the three interpolated BCC time series. OCNM has an average time resolution of 3 years, but to facilitate analysis this record was also re-sampled at the same time points (47-year interval) as BCC by linear interpolation between adjacent data points. For lake sediment records, the Lake Grinnell and Lake Jellybean records have an average resolution of 35 and 22 years, respectively. Both records were re-sampled at a common 35-year interval by linear interpolation. For all time series data δ ( t ), the linear interpolation procedure estimated δ -values for an element t of an evenly spaced time vector based on the two neighbouring measurements δ ( t i ) and δ ( t j ): where t i ≤ t ≤ t j . All interpolation was conducted in Matlab R2012b. Statistical analysis To determine the correlation of paired proxy records, the Pearson coefficient r xy of two time series was calculated as , where n is the sample size, and are the sample means, and S x and S y are the sample s.d. To account for autocorrelation within individual time series, we computed the ‘effective’ sample size [46] : , where r xl and r yl are the autocorrelation at lag l for paired time series. The Student’s t -value for assessing significance was calculated as . The difference between MH and LH δ 18 O values for each record was evaluated using the two-sample t -test [47] with a correction to calculate effective sample numbers accounting for autocorrelation in each record ( n eff = n (1− ρ )/(1+ ρ ), where n is the number observations in a record before correction and ρ is the lag 1 autocorrelation in the time series). Mean values were found to be different with P <<0.01 for all records. The OCNM record has mean δ 18 O values of −8.78±0.18‰ and −9.11±0.23‰ for LH and MH, respectively ( T =4.19, n eff,1 =14, n eff,2 =14, df eff =26). The BCC record has mean values of −6.10±0.08‰ and −5.81±0.09‰ for LH and MH, respectively ( T =−4.52, n eff,1 =4, n eff,3 =3, df eff =5). The Lake Jellybean record has mean values of −19.44±0.36‰ and −19.67±0.26‰ for LH and MH, respectively ( T =2.52, n eff,1 =25, n eff,2 =24, df eff =47). The Lake Grinnell record has mean values of −7.93±0.20‰ and −7.39±0.25‰ for LH and MH, respectively ( T =−4.81, n eff,1 =8, n eff,2 =9, df eff =15). Time series analysis Cross-spectral analysis of each paired δ 18 O time series was performed using the computer package SPECTRUM [48] . We used a Welch-type spectral window, with a number of overlapping (50%) segments ( n seg ) of 5. Considering the 47- (for speleothem) and 35-year (for lake sediment) resolution of our records, we disregard spectral peaks below the Nyquist period of 100 years (0.01 year −1 ). Climate model simulations IsoGSM [34] was run with a horizontal resolution of T62 (about 180 km) and 28 vertical layer to generate the simulations used in this study. We have run three separate sets of simulations. First, for the historical run, that is, 1871–2009, IsoGSM was nudged towards NOAA-20C re-analysis atmospheric data [49] (wind speed, surface temperature and surface pressure) with a spectral nudging technique for large scale (larger than 1,000 km) waves [34] . Second, a LH (present day) simulation was conducted where monthly climatologies of SST and sea-ice distribution for the period 1979–2007 obtained from the Atmospheric Model Intercomparison Project (AMIP) were averaged and used to force the IsoGSM atmosphere. Third, the MH (6 kyr BP) IsoGSM run was performed similar to the LH simulation, but with changes to the surface forcing, orbital parameters and greenhouse gas concentrations. The MH IsoGSM simulation was forced with monthly mean SSTs and sea ice fractions from a 400-year Institute Pierre Simon Laplace atmosphere ocean general circulation model simulation of the MH [50] . We first calculated the SST and sea-ice difference between the MH and pre-industrial simulations by the Institute Pierre Simon Laplace model. Then we added these differences to the SST and sea ice observed for the present-day conditions, as detailed in Risi et al. [35] For the MH IsoGSM simulation, the solar orbital parameters were adjusted (eccentricity=0.018682, precession =0.87 and obliquity=24.105) and the greenhouse gas concentrations were lowered ([CO 2 ]=280 p.p.m., [CH 4 ]=650 p.p.b. [N 2 O]=200 p.p.b., [CFC-11]=0 p.p.t. and [CFC-12]=0 p.p.t.). Both LH and MH simulations were run with a 100-s time step, and neither simulation was spectrally nudged. Both IsoGSM simulations were run for 30 years and the last 20 years were used for analyses. How to cite this article: Liu, Z. et al. Paired oxygen isotope records reveal modern North American atmospheric dynamics during the Holocene. Nat. Commun. 5:3701 doi: 10.1038/ncomms4701 (2014).